Evidence for photochemical production of reactive oxygen species in desert soils The combination of intense solar radiation and soil desiccation creates a short circuit in the biogeochemical carbon cycle, where soils release significant amounts of CO 2 and reactive nitrogen oxides by abiotic oxidation. Here we show that desert soils accumulate metal superoxides and peroxides at higher levels than non-desert soils. We also show the photogeneration of equimolar superoxide and hydroxyl radical in desiccated and aqueous soils, respectively, by a photo-induced electron transfer mechanism supported by their mineralogical composition. Reactivity of desert soils is further supported by the generation of hydroxyl radical via aqueous extracts in the dark. Our findings extend to desert soils the photogeneration of reactive oxygen species by certain mineral oxides and also explain previous studies on desert soil organic oxidant chemistry and microbiology. Similar processes driven by ultraviolet radiation may be operating in the surface soils on Mars. In most ecosystems, microorganisms carry out mineralization of soil organic matter. In desert soils, however, non-biological and biological organic decomposition can be comparable in magnitude. For example, soils from the Atacama Desert, Chile, can oxidize D -alanine and L -glucose at significant rates, although terrestrial organisms do not utilize these enantiomers [1] , [2] . In the Mojave Desert, California, nitrogen oxide (NOy) gases are emitted from desiccated soils [3] at rates comparable to wet soils only if the soils are irradiated by sunlight. In other arid and semi-arid locations, photochemical degradation reportedly accounts for 60% of plant litter decomposition [4] . Studies on the photochemical oxidation of xenobiotic organic carbon (herbicides, insecticides and pesticides) in agricultural soils suggested that 1 O 2 generated by sunlight via the photosensitization of soil organics (and possibly of Ti- and Zn-oxides) to be the main oxidant [5] . The involvement of other reactive oxygen species (ROSs) such as superoxide (O 2 ·− ) and hydroxy ( · OH) radical has been hypothesized as well [6] , [7] , [8] , [9] , [10] , [11] . OH is postulated to result indirectly from the reaction of water with humic substances in the excited triplet state or from degradation of H 2 O 2 by transition metal (Me tr ) cations such as Fe 3+ via a photo-Fenton reaction [10] . However, the photochemical oxidative process and its components are not well understood because of a lack of methods for the detection of the involved ROS in soils and their very short life (1 ns to 1 μs (ref. 12 )). Photogenerated ROS have been identified in laboratory studies on mineral oxides (mainly TiO 2 ) exposed to ultraviolet radiation: atomic oxygen radical anion (O ·− ), ozone radical anion (O 3 ·− , and possibly O 4 ·− ), O 2 ·− and · OH [13] , [14] , [15] . The postulated process in these studies involves ultraviolet-induction of electron mobilization from the oxide surface and its subsequent capture by O 2 to form oxygen radical surface adsorbates [16] . This photo-induced mechanism is also supported by the previously shown generation of O 2 ·− in ultraviolet-exposed plagioclase feldspars [17] . Singlet oxygen ( 1 O 2 ) also has been identified [18] , [19] and may oxidize soil organics via intermediate oxidant products but is not adsorbed on mineral surfaces because it is uncharged. Degradation of organic compounds, mainly via · OH, can be catalysed by the photochemistry (via reduction) of iron (III) species such as Fe(OH) 3 , FeOOH and Fe 2 O 3 (ref. 20 ), besides TiO 2 -mineral oxides. Here we show that metal superoxides and peroxides accumulate in topsoils of the Atacama and Mojave deserts (at mid-summer sunlight irradiance 800–1,000 W m −2 ) at a 10-fold higher level than in a non-arid control site. Moreover, we show that desiccated and aqueous desert soils photogenerate equimolar O 2 ·− adsorbates and · OH, respectively, and also that the reactivity of desert soils is associated with the generation of · OH and the concomitant decrease of soil H 2 O 2 in their aqueous extracts in the dark, possibly via the Fenton reaction due to the presence of Me tr in these soils. For this study, new methods enable the identification of soil O 2 ·− , H 2 O 2 and · OH. These methods are not yet suitable, however, for in situ studies on the seasonal and soil depth-dependent formation rates of detected soil oxidants. Moreover, their specificity restricts the evaluation of only a fraction of the photogenerated ROS involved in the oxidative desert soil chemistry. Although the elucidation of the entire model of desert soil ROS photogeneration is not possible with the available methods, they unveil some key steps as they take place by a photo-induced electron transfer mechanism. In addition, our selected soil desert sites are among the most studied of all the world’s arid locations [1] , [21] , [22] , and thus provide a good basis for considering the environmental effects of aridity on the photochemical production of ROS in desert soils. Detection and stability soil O 2 ·− /peroxides and detection of Me tr We extracted soil metal superoxides as O 2 ·− from desiccated Atacama and Mojave Desert topsoils by acetonitrile and quantified fluorometrically by a modified hydroethidine (HE)-based assay [23] , [24] , and the identity of O 2 ·− and validity of the HE-based assay were verified by a second assay [25] , [26] , a modification of the superoxide dismutase (SOD)-inhibited equimolar reduction of cyt. c by O 2 ·− (Methods, Supplementary Methods ). The methodological baseline for O 2 ·− detection was determined in H 2 O-prewashed and dried soil, a treatment that destroys O 2 ·− by dismutation [12] : Soil metal peroxides (peroxides/hydroperoxides) were quantified upon aqueous extraction as H 2 O 2 (their hydrolysis product shown in reactions 2–4; refs 27 , 28 ): Soil metal peroxides can be present, however, in mixture with metal superoxides that on aqueous extraction also release H 2 O 2 (reaction 1). Thus, the extracted soil H 2 O 2 is the sum of two fractions that can be quantitatively differentiated. The first H 2 O 2 fraction results from equimolar hydrolysis of metal peroxides (equations 2, 3, 4). The second is differentiated from the first because it results from dismutation of × 2 molar metal superoxides (equation 1). Total soil H 2 O 2 extracted from metal superoxides plus peroxides was quantified by a modification of the Fe 2+ -xylenol orange assay (Methods, Supplementary Methods ), using catalase as control [29] . Atacama and Mojave Desert soils contained ∼ 2.0 nmol O 2 ·− g −1 (that is, metal superoxides). 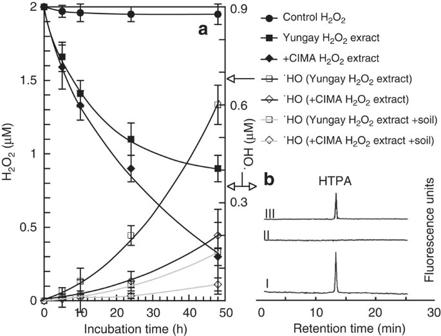Figure 1: Instability of acid-extracted soil H2O2and generation of·OH. Soil H2O2results from the dismutation/hydrolysis of metal superoxides/peroxides, respectively. (a) Decreasing exponential solid line curves depict the change of 10 mM H3PO4-extracted soil H2O2concentration (initially adjusted to 2 μM, and in the absence of the extracted soil) from the Mojave and Atacama +CIMA and Yungay sites (filled rhombs and squares), respectively, versus time, against a 2.0 μM H2O2(in 10 mM H3PO4) control solution (filled circles). Increasing exponential line curves depict the generation (versus time) of·OH in the H2O2extracts from the same Mojave and Atacama sites (open rhombs and squares, respectively) in the absence and presence of soils (solid and dotted lines, respectively). (b)·OH was detected from its reaction with TPA(added to the H2O2extracts at 2 mM) and the equimolar production of the specific fluorescent product HTPA70. HTPA was quantified and identified fluorometrically by HPLC (I, using as controls the·OH scavenger DMSO, II, and pure HTPA, III). Similar data (not shown) were obtained for H2O2extracted from total peroxides from the other tested Atacama and Mojave Desert soil sites. Error bars designate s.d. In contrast, soils from a non-arid control location contained an order of magnitude less concentration of ∼ 0.2 nmol g −1 ( Table 1 ). However, the dry desert soil is conducive to preservation of O 2 ·− , while constantly humid soils are not (because of reaction 1). Even in the deserts, given the extreme labile nature of O 2 ·− , only a small fraction would be stabilized in soils. The Mojave and Atacama Desert soils also contain metal peroxides ( Table 1 ) because the concentration levels of the extracted total soil H 2 O 2 are 5–95 times higher than the H 2 O 2 expected from the (dismutation of) the detected soil metal superoxides. The levels of H 2 O 2 we detected in both Atacama Desert sites are similar to those previously reported [1] . Table 1 Soil metal superoxides, total superoxides/peroxides (H 2 O 2 ) and Fe 3+ . Full size table The detected soil metal superoxides and peroxides were stable even when the desiccated desert soils were heated at 200 °C for 1 h. This agreed with the finding that the desert soils retained ∼ 50% of their initial concentrations in metal superoxides and peroxides after storage for 1year (desiccated in the dark at ∼ 16 °C; data not shown). The extracted H 2 O 2 was not stable through time, however, as almost 50% was destroyed within 1 day in the dark ( Fig. 1a ). This could be because of its decomposition to · OH by co-extracted Me tr via the Fenton reaction [12] , [30] , as supported by the identification of Fe and other Me tr (for example, Cu, Cr, Co, Ni) in these soils ( Tables 1 and 2 ) and the participation of these in the Fenton reaction [31] . Indeed, desert soil H 2 O 2 extracts generated · OH through time ( Fig. 1b , Methods, Supplementary Methods ), the rate of which in the presence of soil decreased by ∼ 6-fold probably because of · OH scavenging by soil organics [32] and/or metal (Me) ions (via the general reaction: · OH+Me n + H 2 O→Me n + OH→Me ( n +1)+ +OH − ; ref. 33 ). Figure 1: Instability of acid-extracted soil H 2 O 2 and generation of · OH. Soil H 2 O 2 results from the dismutation/hydrolysis of metal superoxides/peroxides, respectively. ( a ) Decreasing exponential solid line curves depict the change of 10 mM H 3 PO 4 -extracted soil H 2 O 2 concentration (initially adjusted to 2 μM, and in the absence of the extracted soil) from the Mojave and Atacama +CIMA and Yungay sites (filled rhombs and squares), respectively, versus time, against a 2.0 μM H 2 O 2 (in 10 mM H 3 PO 4 ) control solution (filled circles). Increasing exponential line curves depict the generation (versus time) of · OH in the H 2 O 2 extracts from the same Mojave and Atacama sites (open rhombs and squares, respectively) in the absence and presence of soils (solid and dotted lines, respectively). ( b ) · OH was detected from its reaction with TPA(added to the H 2 O 2 extracts at 2 mM) and the equimolar production of the specific fluorescent product HTPA [70] . HTPA was quantified and identified fluorometrically by HPLC (I, using as controls the · OH scavenger DMSO, II, and pure HTPA, III). Similar data (not shown) were obtained for H 2 O 2 extracted from total peroxides from the other tested Atacama and Mojave Desert soil sites. Error bars designate s.d. 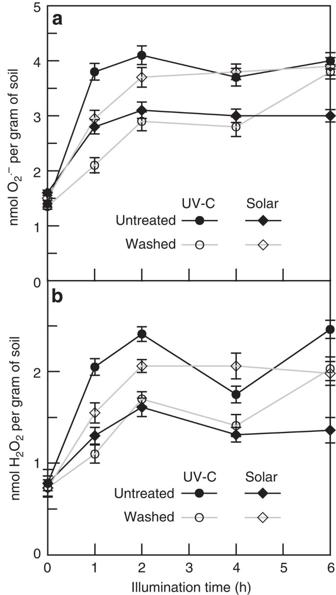Figure 2: Photochemical formation of ROS in desert soils. (a) O2·−was generated in the Mojave Desert +CIMA site (untreated or washed and then dried), which was exposed to solar (natural sunlight) and ultraviolet C irradiation versus exposure time. (b) Generation of total metal superoxides/peroxides (expressed as H2O2) in the same +CIMA site under irradiation conditions as ina. Similar data (not shown) were obtained in the other tested desert/control sites. Error bars designate s.d. Full size image Table 2 Bulk sample chemical analysis. Full size table Photogeneration of soil O 2 ·− and · OH, and mineral analysis ROS were photogenerated (by natural sunlight and ultraviolet C) by desiccated soils. Before exposure soils also were washed to remove any potentially interfering soil inorganics (for example, perchlorates and nitrates known to exist in these deserts [34] , [35] ) and organics (for example, photosensitizers, ROS scavengers; Methods). Soil O 2 ·− and H 2 O 2 (peroxides) concentrations almost doubled or tripled (above baseline; 1.5 and 0.7 nmoles g −1 , respectively) during the first hour of soil irradiation ( Fig. 2 ). A similar trend for O 2 ·− generated on ultraviolet-irradiated plagioclase feldspar minerals has been observed previously [17] . Longer irradiation (up to 6 h) resulted in a concentration plateau for O 2 ·− (similarly for H 2 O 2 ), irrespective of the radiation source (although somewhat higher for the more effective ultraviolet C), which could be due to the saturation of the positively charged sites on the soil surface by the O 2 ·− anion. The concentration of the soil photogenerated O 2 ·− ( Fig. 2a ) was approximately twice that of H 2 O 2 ( Fig. 2b ). This O 2 ·− /H 2 O 2 ratio fits the stoichiometry of the dismutation of O 2 ·− (reaction 1), which indicates that O 2 ·− is the main soil oxidant formed during sunlight/ultraviolet C exposure. Figure 2: Photochemical formation of ROS in desert soils. ( a ) O 2 ·− was generated in the Mojave Desert +CIMA site (untreated or washed and then dried), which was exposed to solar (natural sunlight) and ultraviolet C irradiation versus exposure time. ( b ) Generation of total metal superoxides/peroxides (expressed as H 2 O 2 ) in the same +CIMA site under irradiation conditions as in a . Similar data (not shown) were obtained in the other tested desert/control sites. Error bars designate s.d. Full size image We analysed the mineral substrates potentially involved in the photogeneration of ROS by the Atacama and Mojave Desert and control soils both in the bulk and the clay fractions of the samples (Methods, Supplementary Methods ). All the samples contained plagioclase feldspar with composition that varied from albite to labradorite. Clay minerals were most abundant in the control soil, absent from the Mojave Desert basalt, and found in traces in the remaining samples, in accordance with the Loss On Ignition data in Table 2 . All the soils contain traces of Fe-Ti- and/or Fe-Mn- and/or Fe-oxides and/or Ti-oxides. It has been established that aqueous TiO 2 photogenerate O 2 ·− and · OH [15] , [36] , the latter being photogenerated by aqueous TiO 2 films as well [37] , [38] . The presence in the tested desert soils of Ti-based transition metal oxides prompted us to investigate whether these soils photogenerate · OH under aqueous conditions. Here we show that both Atacama and Mojave soils (0.2 g, prewashed from any soluble inorganic and organic constituents) photogenerate an average of 3.2 nm · OH h −1 ( Fig. 3 ) upon exposure to 180 W m −2 400–700 nm (or 18% that of sunlight) . This rate is proportional to light intensity as well (data not shown), obeying zero-order reaction rate kinetics as in aqueous TiO 2 film photocatalysis [38] . We identified · OH and quantified its rate of photogeneration by a modification of the terephthalic acid (TPA)-based assay [37] , [38] and by the ∼ 15-fold rate decrease caused by the · OH scavenger dimethyl sulfoxide (DMSO; Methods). · OH is not photogenerated by exposing a control H 2 O 2 solution, given that H 2 O 2 is released from metal superoxides/peroxides under aqueous conditions. 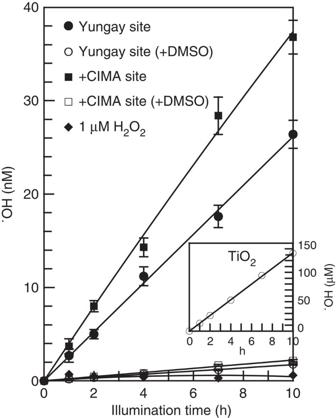Figure 3: Photogeneration of·OH by desert soils under aqueous conditions. Soils (from the Atacama Yungay site and the Mojave +CIMA site) were extensively washed and exposed to light (400–700 nm), against ±100 mM DMSO (·OH scavenger) and an H2O2control, using commercial TiO2(inset) as additional control, given its presence in the tested desert soils. The other tested desert/control sites gave similar data (not shown). Error bars designate s.d. Figure 3: Photogeneration of · OH by desert soils under aqueous conditions. Soils (from the Atacama Yungay site and the Mojave +CIMA site) were extensively washed and exposed to light (400–700 nm), against ±100 mM DMSO ( · OH scavenger) and an H 2 O 2 control, using commercial TiO 2 (inset) as additional control, given its presence in the tested desert soils. The other tested desert/control sites gave similar data (not shown). Error bars designate s.d. Full size image Generation of 3.2 nM · OH in 1 h by 0.2 g soil exposed to 180 W m −2 or 18% that of sunlight corresponds to ∼ 1 nmol g −1 for 1 h exposure to sunlight (see Supplementary Methods ). This is similar to the plateau rate of 1.45 nmol O 2 ·− g −1 that is generated by desiccated (and prewashed) desert soils after exposure to sunlight for 1 h ( Fig. 2a ). This near 1:1 molar O 2 ·− /OH ratio is in agreement with the mechanism of TiO 2 photocatalysis [15] , [36] , which assumes equimolar · OH and O 2 ·− aqueously generated; the latter also being photogenerated in desiccated soils by the same mechanism ( Fig. 4 ). The ratio 1:1.5 deviation from the equimolar ratio could be due to various factors such as the non-aqueous/aqueous generation of additional ROS species (for example, O ·− , O 3 ·− , O 4 ·− ; refs 13 , 14 , 15 ), the not accounted ultraviolet component of natural sunlight, and the possible incomplete trapping of · OH by the assay reagent TPA. Generation of · OH by photodissociated H 2 O 2 , under the employed experimental conditions, may be negligible as shown by the corresponding assay control ( Fig. 3 ). The aqueous photogeneration of · OH by metal oxides in desert soils also was supported by our control experiment with TiO 2 . Tested at a quantity equivalent to its w% concentration in the soils ( Table 2 ), TiO 2 produced · OH at ∼ 13 μM h −1 ( Fig. 3 inset). This ∼ 4,000-fold higher rate compared with the desert soils is because of the very small particle size of TiO 2 (photocatalysis grade, <30 nm in size; ref. 39 ), that results in a highly disordered structure and high specific surface area compared with the natural TiO 2 polymorphs and ilmenite (that is, Fe–Ti oxides) found in the tested soils. 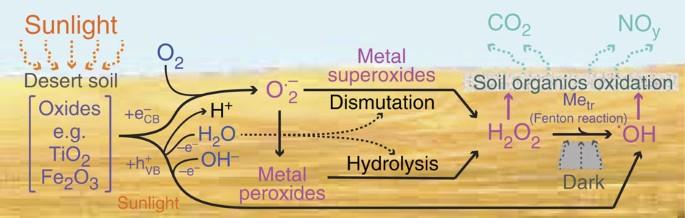Figure 4: Photochemical mechanism of desert soil oxidizing action. Sunlight radiation of soils generates unpaired electrons that convert O2to O2·−. This radical can be initially adsorbed on the surface of soils and stabilized in the long term as metal superoxides and peroxides. These can be converted under aqueous conditions (via dismutation and hydrolysis, respectively) to H2O2, which can be converted subsequently to hydroxyl radical (·OH) in the dark by reaction with reduced soil transition metals (Metr). A second route of·OH generation may involve a single electron abstraction from H2O or OH−by an h+VBhole (see text).·OH (and also H2O2and O2·−, although to a lesser degree as weak oxidants) can then oxidize soil organics possibly to CO2and NOy. Figure 4: Photochemical mechanism of desert soil oxidizing action. Sunlight radiation of soils generates unpaired electrons that convert O 2 to O 2 ·− . This radical can be initially adsorbed on the surface of soils and stabilized in the long term as metal superoxides and peroxides. These can be converted under aqueous conditions (via dismutation and hydrolysis, respectively) to H 2 O 2 , which can be converted subsequently to hydroxyl radical ( · OH) in the dark by reaction with reduced soil transition metals (Me tr ). A second route of · OH generation may involve a single electron abstraction from H 2 O or OH − by an h + VB hole (see text). · OH (and also H 2 O 2 and O 2 ·− , although to a lesser degree as weak oxidants) can then oxidize soil organics possibly to CO 2 and NOy. Full size image Superoxide radical is photogenerated in desert soils ( Fig. 2a ) and stabilized initially as surface-saturating desiccated anionic adsorbate, given that it is the least reactive hence the most stable species formed by ultraviolet exposure [17] . Long-term diffusion of O 2 ·− may be the subsequent stabilization process, as metal superoxides and peroxides were detected in the Atacama and Mojave Desert soils. This is in agreement with the finding that the average concentration of metal superoxides in a basalt rock (pulverized) from the Mojave Desert +CIMA field is similar to their concentration in the surrounding sand ( Table 1 ), suggesting a long-term O 2 ·− diffusion inside basalt rocks. Such diffusion through soils does not occur within the short irradiation period used in our and similar studies (with labradorite), since this is considered geologically very short [17] . In general, the main conditions under which stable O 2 ·− is formed on the surface of metal oxides and zeolites are (i) photoinduced electron transfer, (ii) direct surface-oxygen electron transfer, (iii) surface intermolecular electron transfer and (iv) the decomposition of H 2 O 2 (ref. 40 ). The photo-induced electron transfer mechanism ( Fig. 4 ) could involve ejection from transition or non-transition metal oxides (for example, TiO 2 , Fe 2 O 3 (ref. 20 ), or ZnO (ref. 41 ), respectively) of an electron (e − CB ) into its CB (conduction band) from its valence band (VB), and its transfer to O 2 with concomitant generation of O 2 ·− , leaving a positively charged hole (h + VB ) at the band edge of the VB. In addition to O 2 ·− , an adsorbed · OH may be formed on the oxide surface, from an e − abstracted by the h + VB hole from H 2 O or OH − (refs 15 , 36 , 40 , 42 ). Nonetheless, O 2 may not be the only acceptor of the photogenerated single electrons, as 1 O 2 also possesses sufficient one-electron reduction potential to form O 2 ·− (ref. 43 ). Then, the photogenerated O 2 ·− could be adsorbed on the surface of minerals where it could saturate their positively charged sites. In the long term, O 2 ·− may migrate via diffusive transport to greater depths in the soils, where it may stabilize as metal superoxides and peroxides ( Table 1 ). Metal superoxides/peroxides are better preserved (protected from dismutation/hydrolysis, respectively) in desiccated soils than in soils containing water [42] . This, in turn, depends on the clay mineral composition. Swelling clay minerals (smectite and vermiculite), that were more abundant in the control site soil, readily adsorb H 2 O molecules, thus contributing to greater water adsorption [44] and possibly to lower stability of O 2 ·− and metal peroxides. This assumption could explain the observed 10-fold lower concentration of metal superoxides and the much lower concentration of metal peroxides in the control soil compared with the desert soils ( Table 1 ). Moreover, the presence of albite and labradorite plagioclase in the Atacama and Mojave Desert soils, respectively, is in agreement with the previously proposed ultraviolet-induced mechanism of O 2 ·− generation by these minerals [17] , [42] . The same mechanism might also apply for the albite-bearing control site soil. Also, metal superoxides and peroxides may be continuously photogenerated in all soils because TiO 2 , Fe-oxides and Fe-Ti-oxides—present in the tested soils and typical of desert soils [45] —are known to be involved in the photogeneration process of O 2 ·− (refs 13 , 14 , 15 , 17 , 36 ). In addition to Ti (in Ti- and/or Fe-Ti-oxides) as well as Fe and Mn (in Fe- and/or Mn-oxides either free or impurities in silicate minerals), the long-term stabilization process for adsorbed soil O 2 ·− as metal superoxides and peroxides also may involve (besides Ti [46] ) the exchangeable metals Ca, Na and K that are present in smectite. Specifically, O 2 ·− may be stabilized as (i) metal superoxides such as KO 2 and NaO 2 , (ii) metal peroxides such as Na 2 O 2 , CaO 2 , K 2 O 2 and TiO 3 ·2H 2 O and TiO 2 ·2H 2 O (both less water soluble) that are usually formed by the reaction of the metal with H 2 O 2 and (iii) metal hydroperoxides such as NaOOH, (KOOH) 2 ·3H 2 O and Ti(OH) 3 OOH) [27] , [28] . The photochemical production of O 2 ·− as soil adsorbate and stabilized as metal superoxides/peroxides could explain the reactivity of desert soils with organics ( Fig. 4 ) under several considerations. Soil H 2 O 2 (for example, aqueously generated via reactions 1–4) can decompose carbohydrates to formic acid and ultimately to CO 2 (ref. 47 ). The release of NOy from the Mojave Desert soil [3] and N 2 O from the Atacama Desert soil [48] ) could have resulted from · OH by the following mechanism: · OH can oxidize amino acids with ammonia as a byproduct. Ammonia can be further oxidized by · OH to amidogen radical [49] , that can subsequently react with O 2 to form nitric oxide radical ( · NO), dioxide radical ( · NO 2 ) and N 2 O (refs 49 , 50 , 51 ). Hydroxyl radical can be generated from H 2 O 2 (the product of dismutation/hydrolysis of metal superoxides/peroxides, respectively) either by the Fenton reaction (5) catalysed by Me tr or by O 2 ·− via the Me tr -catalysed Haber–Weiss reaction (6) [30] : The Fenton mechanism is considered probable because Me tr (Fe 3+ and trace elements Cu, Cr, Co and Ni) were identified in Mojave and Atacama Desert soils ( Tables 1 and 2 ). Me tr might exist in the desert soils in their reduced and/or oxidized form and can participate in the Fenton reaction (5) with their reduced form directly. For example, Fe 2+ might occur as interlayer species such as the Fe 2+ -aquo complex in the 2:1 clay minerals [52] . Also Fe 3+ may participate in the Fenton reaction indirectly after its reduction by H 2 O 2 (ref. 30 ) or O 2 ·− (O 2 ·− +Me tr n +1 → Me tr n +O 2 ; the sum of this reaction with the Fenton reaction 5 is the Me tr -catalysed Haber–Weiss reaction 6; ref. 12 ). Therefore, Me tr can convert the weak oxidants H 2 O 2 and O 2 ·− to the highly reactive · OH. We showed that the instability of the Atacama and Mojave Desert soil metal superoxides/peroxides (as H 2 PO 4 -extracted H 2 O 2 ) in the dark is associated with the production of · OH ( Fig. 1 ). The possible involvement of the Fenton reaction mechanism can be implied by the concurrence of the higher (threefold) production of · OH in Atacama (Yungay site) over Mojave (+CIMA site) with the higher concentration of Me tr (four and twofold higher in Cu and Co), respectively ( Table 2 ). H 2 O 2 could be destabilized by other factors such as alkaline pH (via the hydrolysis reaction: 2H 2 O 2 →2H 2 O+O 2 ; ref. 53 ). However, this is not a likely scenario given the stabilizing effect of phosphates and acidic pH on H 2 O 2 (ref. 54 ), with the latter confirmed by the relative stability of a control H 2 O 2 solution in 10 mM H 3 PO 4 ( Fig. 1a ). Therefore, the identification of · OH in the Atacama aqueous soil extracts ( Fig. 1a ) could explain the previous observation of the oxidation (to CO 2 ) of sodium formate and aqueous mixtures of chiral sodium alanine and glucose after incubation for several days with Atacama Desert soil even in the dark, albeit at a slower rate [1] . The reactivity of the Atacama Desert soils with organics in the dark may not proceed by direct involvement of 1 O 2 , as its lack of charge would hinder its adsorption on the surface of soils. Moreover, non-light-induced abiotic oxidation of organics also may be involved in desert soils because the process has shown that Mn-oxides and Fe-oxides/hydroxides common in desert soils (and in the tested ones, Table 2 ) could cause oxidation of organics (for example, 17beta-estradiol [55] ) and aromatic amines [56] . Similarly, perchlorates (present in both Atacama and Mojave Deserts [34] , [35] ) could be potential oxidants of soil organics [57] , [58] , [59] . The oxidation of soil organics by photogenerated ROS may be a continuous process given that Me tr are ubiquitous in all soils. O 2 ·− may represent a fraction of the ROS produced in photo-irradiated desert soils, however. Another ROS could be 1 O 2 because it is generated—and oxidizes organics—by photo-irradiated minerals such as MgO, Al 2 O 3 and SiO 2 (refs 18 , 19 , 60 ), which are common in desert soils and also found in the tested soils ( Table 2 ). Moreover, 1 O 2 could be formed directly by reaction of O 2 ·− with H 2 O 2 (refs 61 , 62 ), and possibly by the decomposition of light-generated O 2 ·− on irradiated surface soils [18] . In addition, 1 O 2 can form O 2 ·− because it possesses the required one-electron reduction potential (+0.65 V at pH 7.0), while its two-electron reduction could generate H 2 O 2 (ref. 43 ). Therefore, photogeneration of O 2 ·− from 1 O 2 could have been possible under non-aqueous conditions as long as it involves a highly reactive single electron photo-ejected from soil minerals or donated by soil organic photosensitizers. The present study also showed that O 2 ·− is photogenerated by desert soils ( Fig. 2a ). O 2 ·− is generated at similar levels even by soils prewashed before exposure from polar inorganic and polar/non-polar organic soil constituents, suggesting a mechanism not involving photosensitization and the involvement of perchlorates. These prewashed soils also photogenerated · OH under aqueous conditions ( Fig. 3 ) and at a near 1:1 molar rate ratio with the O 2 ·− that is generated (in the 1st hour) by sunlight-exposed desiccated soils ( Fig. 2a ), in agreement with the mechanism for TiO 2 photocatalysis [15] , [36] . The same mechanism also could apply for the desert soils ( Fig. 4 ) since they contain transition metal oxides such as TiO 2 and Fe-Ti-oxides ( Table 2 ). Moreover, the photo-catalytic generation of · OH by aqueous desert soils could provide a light-based mechanism for their reactivity with organics. This would involve the photo-catalytic ejection of an electron from metal oxides (to generate O 2 ·− by dissolved O 2 ) and the subsequent abstraction of an electron by the resulting h + VB hole from H 2 O or OH − (resulting also from H 2 O via reaction with a bridging-oxygen atom [15] ). Then, · OH (and H 2 O 2 to a lesser degree) could oxidize soil organics to CO 2 and NOy. The photogenerated ROS detected in desert soils also may explain the ionizing radiation resistance of certain desert bacteria—notably Deinococcus radiodurans and Chroccocidiopsis —that can withstand extraordinarily high levels of ionizing radiation [63] . Radiation resistance is regarded as a proxy for desiccation resistance [63] . Ionizing radiation also produces reactive oxidants similar to photochemical oxidants [64] . Thus, the ability to withstand photochemical oxidants might explain the resistance of desert bacteria to radiation. Finally, an extreme example of this soil oxidant chemistry appears to take place on Mars. The oxidative reactivity of the Martian soil as measured by the Viking Biology Experiments (and exhibited on the organics of a certain nutrient by releasing O 2 and CO 2 (refs 65 , 66 )), requires a mix of oxidants in the soil including oxidants capable of destroying organics [57] , [67] . Production of O 2 ·− by the photo-induced transition metal oxide surface-O 2 electron transfer mechanism has been suggested [17] . Other alternative potential pathways may involve (i) photogeneration of ROS on mineral substrates (for example, plagioclase) that can generate O 2 ·− from adsorbed O 2 on TiO 2 and (ii) photoactive on Mars Fe-oxides such as hematite being analogous to TiO 2 in surface catalysis [42] . The source of O 2 needed for the photogeneration of O 2 ·− in Martian topsoil under an O 2 -depleted atmosphere, however, has not been elucidated. It could be that O 2 might have been released by perchlorate (given its abundance on Mars [68] , [69] ) on exposure to cosmic radiation. This is supported by the generation of O 2 by perchlorate exposed to gamma rays in a CO 2 atmosphere [57] . Nonetheless, the buildup of soil ROS oxidants on Mars would be less impeded by liquid water than even the driest desert on Earth. Accumulated metal superoxides and peroxides were detected in soils from the Atacama (hyper-arid) and Mojave (arid) deserts. Moreover, desiccated desert soils photogenerate O 2 ·− at saturation levels, followed by long-term stabilization by diffusion as soil metal superoxides and peroxides. Desert soils photogenerate · OH under aqueous conditions. The photogeneration of O 2 ·− by desiccated or aqueous soils may proceed via capture by O 2 of a single electron that is photo-ejected from metal oxides (for example, TiO 2 /Fe 2 O 3 detected in the tested soils). The resulting h + VB hole in H 2 O-wetted soil metal oxides can, then, abstract a single electron from H 2 O or OH − and generate · OH. Moreover, aqueous desert soil metal superoxides/peroxides are converted (by dismutation/hydrolysis, respectively) to H 2 O 2 , the observed instability of which in the dark concurs with the generation of · OH, possibly via the Fenton reaction due to the presence in these soils of Me tr . The generation of · OH, in the dark (via the Fenton reaction) and by photocatalysis could explain the abiotic oxidation of organics by desert soils, with H 2 O 2 and O 2 ·− acting as weak oxidants. Similar ultraviolet-induced processes may take place in the topsoils of Mars. Samples and reagents Full details of sample collection and treatment are available in the Supplementary Methods section, with details of the reagents used. HE-based soil O 2 ·− assay Assay principle and other supporting control experiments are described in full in the Supplementary Methods . Reagent solutions 100% alkaline acetonitrile . It is made by mixing 100% acetonitrile (ACN) with 0.1 M NaOH at a 100:1 ratio. At this NaOH proportion (it mixes almost completely as it leaves a small aqueous droplet in the bottom of the tube, resulting in ∼ 99% ACN) and higher, the resulting ACN alk solvent is saturated with hydroxyl ions, reaching a stable pH 8–8.5. For the pH measurements a Sentron Argus-type pH Meter was used, equipped with a non-glass Hot-Line electrode (Sentron, The Netherlands). 100 mM CE . It is prepared by dissolving 186 mg dicyclohexano-18-crown-6 ether (CE) in 5 ml ACN alk . Prepare fresh, keep at 4 °C. Caution: accurate pipetting of the reagent is required. Soil O 2 ·− ACN alk -CE extraction solutions . Solution ACN alk -CE (0.2 mM) is prepared by mixing 29.94 ml ACN alk with 60 μl 100 mM CE. This standard solution is designated also as ACN alk -CE. ACN alk solutions containing other CE concentrations can be prepared from the 100% ACN alk and 100 mM CE stocks. For example, ACN alk -CE (1 mM) solution is made by mixing 29.7 ml ACN alk with 0.3 ml 100 mM CE. The ACN alk -CE extraction solutions should be prepared fresh, and kept in an airtight and light-protected glass container at 4 °C. 0.5 mM HE . Prepare fresh (and kept at 4 °C, protected from light) by dissolving 1.2 mg HE in 7.5 ml ACN alk -CE (0.2 mM) solution. Caution: accurate pipetting of the reagent is required. 50 mM HCl . Prepare by diluting × 240 (with ddH 2 O) the concentrated 37% HCl (or 12 M). Caution: accurate pipetting of thr reagent is required. 1 M Tris-base, pH 8.0 . Caution: accurate pipetting of the reagent is required. Protocol Soil samples were treated as follows: 1 g soil is placed in a 15-ml plastic centrifuge tube (with conical bottom) with 2.5 ml ACN alk or ACN alk -CE (for example, 0.2 mM) and mixed by shaking for 2–3 min at room temperature (RT; to extract O 2 ·− ), and the soil is removed by precipitation (or filtration). The supernatants are diluted appropriately with ACN alk -CE to set the CE concentration in the ACN alk extract to final 0.2 mM and are kept capped in an ice-water bucket. NOTES: I. Soil metal superoxides can be extracted effectively by an ACN alk -CE solution. Testing various concentrations of CE (for example, 0.2, 1 mM) in the ACN alk extraction solution allows the determination of the optimum CE concentration for solubilizing the maximum quantity of soil metal salts of O 2 ·− . This can be tested by extracting soil O 2 ·− with ACN alk mixed with various CE concentrations, to determine a minimum CE concentration above which the extracted O 2 ·− g −1 soil is constant. II. For extracting soil-adsorbed O 2 ·− the ACN alk extraction solution does not need the presence of CE and the ACN alk solution can be used alone. However, ACN alk may also extract soil metal superoxides although not as effectively as being in mixture with CE. The ACN alk -CE supernatants from the preceeding step are split in two halves (in two 1.5-ml microcentrifuge tubes), one designated ‘sample’ (S) and the other ‘blank’ (B), which are centrifuged at 12,000 g for 3 min at RT to remove any soil remnants. Then, 880 μl clear supernatant from each half tube are transferred in new tubes to each of which 80 μl 0.5 mM HE are added (40 μM final in the assay). NOTES: I. For this step, sample/blank tubes are kept in an ice-water bath. II. If using quartz micro-cuvette holding a sample volume 0.3–0.5 ml, (cuvette dimensions 45 × 4 × 4, mm with the Shimadzu RF-1501 spectrofluorometer), the total sample volume required can be minimized to ∼ 1 ml (0.45 ml per S and B), which results in halving the volumes of the reagents added in this and in the subsequent two steps. Thereafter, the following alternative Procedures A and B can be followed: Procedure A: to the B and S tubes, 20 μl 50 mM CE and 20 μl ACN alk -CE (0.2 mM) are added, respectively, followed by the addition in both tubes of 20 μl 50 mM HCl (1 mM H + concentration in the final assay mixture) and mixing by inversion up to 1 min. For preparing the assay reagent blanks, in each of the two microcentrifuge tubes 880 μl ACN alk -CE (0.2 mM) and 80 μl 0.5 mM HE are added, followed by the addition in one tube of 20 μl 50 mM CE and 20 μl 50 mM HCl (designated R CE -1 mM ) and in the other tube of 20 μl ACN alk -CE (0.2 mM) and 20 μl 50 mM HCl (designated R CE-0.2 mM ). NOTES: I. In the S tube, HE reacts with O 2 ·− (the reaction requires at least 0.5 mM H + ) and forms the fluorescent product 2-hydroxy ethidium (2-OH-E + ; at molar stoichiometric ratio O 2 ·− /2-OH-E + =2/1) at 0.2 mM CE, while in the B tube, this reaction is inhibited by the inclusion of 1 mM CE. II. For the reaction of HE with O 2 ·− in 1 mM HCl to take place, the pH of the assay mixture must be acidic (pH 1.5–2). Possible alkalinity of soil may change this pH, therefore, a test of the assay mixture pH must be performed and if needed the final concentration of HCl can be adjusted appropriately to bring the assay pH to 1.5–2. III. This step and the subsequent two steps are performed as soon as possible to minimize the possible oxidation of HE by any extracted soil constituents. After the 1-min incubation period, the assay mixtures in the S, B, R CE-1 mM and R CE-0.2 mM tubes are mixed with 10 μl 1 M Tris by brief vortexing (to adjust the assay mixture pH to ∼ 8), centrifuged at 12,000 g for 1 min and the resulting supernatants are collected for fluorescence measurement. The fluorescence units (FUs) of the S, B, R CE-0.2 mM and R CE-1 mM supernatants are measured at ex/em 505/580 nm (designated FU S , FU B , FU RCE-0.2 mM and FU RCE-1 mM , respectively). From these FU, the net FU of 2-OH-E + is calculated from the following formula: . NOTES: I. To verify that the net corresponds to the concentration of the extracted O 2 ·− , various dilutions of the ACN alk -CE supernatants (derived in the first two steps of the Assay Protocol) should be tested (as in this and the previous two steps in Procedure A) and only those dilutions resulting in proportional values will be used for determining the final average value. II. The FU RCE-0.2 mM and FU RCE-1 mM values can be kept as low as possible by setting the HE final concentration in the assay (see second step in the Assay Protocol) at low levels (for example, 20–40 μM HE), given that O 2 ·− is quite stable in the ACN alk extraction solvent. The FU RCE-0.2 mM −FU RCE-1 mM value is in the order of 50 FU. Much higher values suggest an excessive autoxidation of HE, and a fresh HE stock solution (see Assay Reagent Solutions) should be used. III. In case FU S <FU B , the soil extract may contain a soil constituent, which in the presence of 1 mM CE (in tube B) oxidizes HE to E + . In this case, the alternative Procedure B is followed. Procedure B: to the B and S tubes, 40 and 20 μl ACN alk -CE (0.2 mM) are added, respectively, followed by the addition in the S tube of 20 μl 50 mM HCl (1 mM H + concentration in the final assay mixture) and mixing by inversion up to 1 min. For preparing the assay reagent blanks, in each of the two microcentrifuge tubes 880 μl ACN alk -CE (0.2 mM) and 80 μl 0.5 mM HE are added, followed by the addition in one tube of 20 μl ACN alk -CE (0.2 mM) and 20 μl 50 mM HCl (designated R HCl-1 mM ) and in the other tube of 40 μl ACN alk -CE (0.2 mM) (designated R HCl-0 mM ). NOTES: I. In the S tube, HE reacts with O 2 ·− (the reaction requires at least 0.5 mM H + ) and forms the fluorescent product 2-OH-E + (at 0.2 mM CE), while in the B tube, this reaction does not take place (also in the presence of 0.2 mM CE) because HCl is absent. II. For the reaction of HE with O 2 ·− in 1 mM HCl to take place, the pH of the assay mixture must be acidic (pH 1.5–2). Possible alkalinity of soil may change this pH, therefore, a test of the assay mixture pH must be performed, and if needed the final concentration of HCl can be adjusted appropriately to bring the assay pH to 1.5–2. III. This step and the subsequent two steps are performed as soon as possible to minimize the possible oxidation of HE by any co-extracted soil constituents. After the 1-min incubation period, the assay mixtures in the S, B, R HCl-1 mM and R HCl-0 mM tubes are mixed with 10 μl 1 M Tris by brief vortexing (to adjust the assay mixture pH to 7–8), centrifuged at 12,000 g for 1 min and the resulting supernatants are collected for fluorescence measurement. The FU of the S, B, R HCl-0 mM and R HCl-1 mM supernatants are measured at ex/em 505/580 nm (designated FU S , FU B , FU RHCl-0 mM and FU RHCl-1 mM , respectively). From these FU, the net FU of 2-OH-E + is calculated from the following formula: . NOTES: I. To verify that net corresponds to the concentration of the extracted O 2 ·− , various dilutions of the ACN alk -CE supernatants (derived as in the first two steps of the Assay Protocol) should be tested (as in this and the previous two steps in Procedure B) and only those dilutions resulting in proportional values will be used for determining the final average value. II. The FU RCE-0.2 mM and FU RCE-1 mM values can be kept as low as possible by setting the HE final concentration in the assay (see second step in the Assay Protocol) at low levels (for example, 20–40 μM HE). The FU RHCl-1 mM −FU RHCl-0 mM value should be in the order of 100 FU. Much higher values suggest an excessive autoxidation of HE, and a fresh HE stock solution (see Assay Reagent Solutions) should be used. To convert the net value to the concentration of 2-OH-E + (and subsequently of O 2 ·− ) in the assay mixture volume (1 ml, in this case), the spectrofluorometer in use must be calibrated with known concentrations of 2-OH-E + by determining the fluorescence extinction coefficient of 2-OH-E + (FEC 2-OH-E + , expressed in FU per 1 μM −1 2-OH-E + ) as follows. The FEC 2-OH-E + is determined in final 97% ACN (same as the ACN final concentration in the assay reaction mixture) for the spectrofluorometer (set at high sensitivity) and quartz cuvette in use in this study, as follows: from a synthetic 2-OH-E + stock solution (see Supplementary Methods ) of known concentration, 1 μM 2-OH-E in 1 ml ACN alk (or 1 ml ACN alk -CE extraction solution) is prepared in a 1.5-ml microcentrifuge tube, to that 2 μl ddH 2 O and 30 μl 0.33 M Tris solution are added, and vortexed, and centrifuged at 12,000g for 1 min. Similarly is treated a reagent blank, which is prepared with 1 ml ACN alk (or 1 ml ACN alk -CE extraction solution), containing 2 μl ddH 2 O and 30 μl 0.33 M Tris solution. FEC 2-OH-E + is determined by measuring the FU value of the clear 1 μM 2-OH-E + supernatant (at ex/em 505/580 nm) and subtracting from this value the FU of the clear supernatant of the blank. Having determined in the preceeding step, and given the molar stoichiometric ratio O 2 ·− /2-OH-E + =2/1, the (determined three steps before) is converted to a μM concentration of 2-OH-E + (in the assay mixture volume) and then to μM O 2 ·− by the formula (see derivation in Supplementary Methods ): Finally, the μM O 2 ·− (extracted from a known soil quantity) are converted to nmoles O 2 ·− g −1 soil. Assay sensitivity Applying the protocol on 1 g soil, extracted in 1 ml ACN alk -CE solution by filtration (to recover a ∼ 1.0 ml ACN alk -CE extract), with an assay reaction volume 0.5 ml (containing 0.44 ml ACN alk -CE extract) and a minimum net , the theoretical assay sensitivity (using the above formula) is=200 × 2/1300= ∼ 0.3 μM O 2 ·− (in the assay reaction mixture, or 0.34 nmoles in 1.0 ml ACN alk -CE extract, or 0.34 nmoles g −1 soil). SOD-inhibited reduction of cyt. c -based soil O 2 ·− assay Protocol . Soil samples were mixed with a minimum 0.3 ml O 2 -degassed ACN alk -CE (0.2 mM) per gram of soil by shaking for 2–3 min at RT. This proportion achieves the maximum concentration of O 2 ·− extracted in a minimum solvent volume. Then, ∼ 0.5 g batches of this soil/ ACN alk -CE slurry were placed in centrifuge tube filters fitted to a 1.5-ml microcentrifuge collection tube, centrifuged at 15,000 g for 5 min and the O 2 ·− /ACN alk -CE eluents of all the batches were combined and used in the following step. NOTE: In this step and in subsequent steps, all the reagents used should be O 2 -degassed as in two steps before. Having established the molar stoichiometric ratio 1:1 of O 2 ·− to cyt. c red up to a final 40% ACN alk -CE (see Supplementary Methods ), the maximum ACN alk -CE solvent volume for the recovery of O 2 ·− from any soil sample is 0.4 ml. This volume is sufficient for the control if ∼ 0.5-volume capacity cuvettes are used. Given that the minimum proportion of ACN alk -CE extraction volume/soil weight is ∼ 0.3 ml per 1 g, the maximum amount of soil that this assay can extract for measuring accurately the concentration of O 2 ·− in a 0.4 ml extract is 1.3 g. Therefore, 1.3-g soil samples were used extracted in 0.4 ml ACN alk -CE, and were diluted with 100% ACN alk -CE to 0.8 ml (unless a smaller than 1-ml spectrophotometer cuvette is used). A 0.4 ml portion of the clear ACN alk -CE-O 2 ·− extract (after centrifugation at at 15,000 g for 5 min) was mixed with 0.6 ml 50 mM phosphate buffer, pH 7.8, containing 26.7 μM cyt. c ox (final 16 μM). Its absorbance was measured at 550 nm against a reagent blank (0.4 ml ACN alk -CE plus 0.6 ml 50 mM phosphate buffer, pH 7.8) and also against the following SOD blank: It consists of the remaining 0.4-ml portion of the ACN alk -CE extract, mixed with 0.6 ml 50 mM phosphate buffer, pH 7.8, containing 26.7 μM cyt. c ox and 3.3 units SOD (or SOD added before the addition of cyt. c ox ). If O 2 ·− is present in the 0.4 ml ACN alk -CE extract the assay will identify it from the SOD-inhibited reduction of cyt. c ox . Competing with cyt. c ox , SOD will reduce or eliminate the concentration of O 2 ·− by dismutation. This blank also quantifies possible soil contaminants that may cause chemical reduction of cyt. c ox and/or absorb at 550 nm. Then, the Δ A 550 nm (absorbance of the sample minus absorbance of the SOD blank) is converted nmoles of cyt. c red , which correspond to equimolar O 2 ·− derived from the standard curve of cyt. c red versus O 2 ·− concentration (see Supplementary Methods ). The sensitivity of the assay is ∼ 0.5 nmoles O 2 ·− (or 0.5 μM in the ACN alk -CE/phosphate buffer assay mixture). NOTE: The 0.4 ml of the ACN alk -CE-O 2 ·− soil extract should be rapidly mixed with the 0.6-ml phosphate-buffered cyt. c ox in the spectrophotometer cuvette and its peak absorbance immediately measured as it rapidly decreases due to the reoxidation of cyt. c red . Assay for soil total metal superoxides/peroxides and Fe 3+ Reagent solutions . FOX (Ferrous Oxidation in Xylenol orange) assay reagents. In a plastic vial (glass vials may leak Fe 3+ ), 3.644 g sorbitol (final 2 M, and in assay reaction 0.1 M) and 15.2 mg xylenol orange are dissolved (for about 30 min) in 7.6 ml 0.66 M HClO 4 (final 0.5 M, and in assay reaction 25 mM). Then, any non-dissolved matter is removed by centrifugation (or by filtering), the resulting supernatant is split in two halves (5 ml each), and one half is the FOX-Fe 2+ reagent. To the other half, 7.9 mg ferrous ammonium sulfate are dissolved, resulting in the FOX+Fe 2+ reagent. Both the reagents are prepared fresh. 0.1 M EDTA stock . It is prepared in ddH 2 O. EDTA is a Fe 3+ chelator, and is used here as blank for the estimation of soil Fe 3+ . Standard curves H 2 O 2 (0–2 μM) standard curve . It is made with a 4 μM H 2 O 2 solution (in 10 mM phosphate buffer, pH 6.5) prepared from a 5 mM H 2 O 2 working stock, which is made from the concentrated 30% H 2 O 2 using the H 2 O 2 molar extinction coefficient at 240 nm ( ɛ 240 =43.6 M −1 cm −1 ). The reagents are mixed as presented in the following box: Each tube is then incubated for 30 min at RT after which the absorbance at 560 nm ( A 560 nm ) of each of the assay reaction mixtures in tubes 0–2 is measured. The net A 560 nm value of tubes 0.2–2 is calculated by subtracting from their A 560 nm value the A 560 nm value of tube 0 (the blank). Then, the standard curve is drawn by plotting the 0–2 μΜ (or nmoles) H 2 O 2 against their corresponding net A 560 nm values. NOTE: With 10 mM phosphate, pH 6.5, as H 2 O 2 /sample solvent, the final 25 mM perchloric acid in the assay achieves assay reaction pH ∼ 1.8. At these conditions, the assay achieves its highest, for H 2 O 2 , molar extinction coefficient ∼ 250,000 M −1 cm −1 ). With unbuffered samples (that is, in H 2 O), the final concentration of perchloric acid in the assay should be 15.5 mM (in H + ), which corresponds to the optimal assay pH 1.8. Fe 3+ (0–12 μM) standard curve It is made from a 20 μM Fe 3+ stock solution (in 10 mM phosphate buffer, pH 6.5). The reagents are mixed as presented in the following box: Each tube is then incubated for 30 min at RT after which the absorbance at 560 nm ( A 560 nm ) of each of the assay reaction mixtures in tubes 0–12 is measured. The net A 560 nm value of tubes 1–12 is calculated by subtracting from their A 560 nm value the A 560 nm value of tube 0 (the blank). Then, the standard curve is plotted as 0–12 μΜ (or nmoles) Fe 3 against their corresponding net A 560 nm values. Protocol Soil samples were treated as follows: 1 g soil (placed in a capped 15-ml plastic centrifuge tube) was extracted in (for example, 1–4 ml) 10 mM H 3 PO 4 for 2 min by gentle inversion and the soil extract was collected by centrifugation at 5,000 g for 5 min. NOTE: Extraction of the Mojave and Atacama soil samples with 10 mM H 3 PO 4 resulted in pH ∼ 6.5 of the soil H 2 O 2 extract. The soil extract (its pH is adjusted to ∼ 6.5 with 0.1 M NaOH/HCl if needed) was treated with the assay reagents (in 1.5-ml microcentrifuge tubes) shown as presented in the following box: After mixing, the ST1, ST2, ST3, ST4, RB1 and RB2 tubes are incubated for 30 min at RT. NOTE: For higher accuracy, ST1, ST2, ST3 and ST4 mixtures are preferably made each in triplicates from three different soil extract dilutions, while RB1 and RB2 are made in triplicates. The corresponding A ST1 , A ST2 , A ST3 , A ST4 , A RB1 and A RB2 absorbance values are recorded at 560 nm, and their triplicate averages are then entered in the following equations to calculate the corresponding net A 560 nm for soil H 2 O 2 and Fe 3+ , which are then converted to H 2 O 2 and Fe 3+ concentrations (from the corresponding standard curves), expressed per g soil: Instability of aqueous desert soil superoxides/peroxides To test whether the instability of soil H 2 O 2 extracts (from total metal peroxides) during various incubation intervals concurs with the generation of · OH radicals, these were trapped in the H 2 O 2 extracts by TPA and the resulting specific fluorescent product 2-hydroxyl terephthalate (HTPA) was isolated and quantified by the following procedured developed for this study. Procedure: Soil H 2 O 2 extracts were analysed for stability and · OH generation versus extract incubation time (0–48 h) in the absence (A) and presence (B) of the extracted soil. Specifically, H 2 O 2 was extracted from two 1-g soil samples (per incubation time interval) after each was mixed with 4 ml 10 mM H 3 PO 4 for 5 min at RT, followed by centrifugation at 4,200 g for 3 min. The H 2 O 2 extract in the isolated supernatant (in the absence of the soil precipitate) was kept for treatment A and that in the upper aqueous phase (in the presence of the soil precipitate) was kept for treatment B. Stability of H 2 O 2 in extract samples from treatment A was measured as the remaining H 2 O 2 concentration after certain incubation time intervals (up to 48 h) at RT, using as control a solution of 2 μM H 2 O 2 in 10 mM H 3 PO 4 (made from the 30% H 2 O 2 , the preparation of which is described in the H 2 O 2 standard curve presented in the Methods section ‘Assay for soil total metal superoxides/peroxides and Fe 3+ ’). The concentration of H 2 O 2 was measured as described in the Methods section ‘Assay for soil total superoxides/peroxides and Fe 3+ ’. More experimental details are also presented in the legend of Fig. 1 . To measure the generation of · OH in the extracts of treatments A and B, they were both brought to 2 mM TPA (from a 100 mM TPA stock made by dissolving 115 mg TPA in 1.4 ml 1 M NaOH and then mixing with 1.4 ml 50 mM phosphate buffer, pH 7.4, readjusted with 1 M HCl and ddH 2 O to final 7 ml) and incubated at RT in the dark for the selected time intervals. As control, corresponding soil extracts were also incubated with 100 mM DMSO), an · OH scavenger. After each incubation period, 0.9 ml of the soil extracts for treatments A and B were mixed with 9 μl 10 M NaOH (to ensure deprotonation of HTPA) and washed with an equal volume ethyl acetate–ethanol (2:1) by vortexing, followed by centrifugation at 4,200 g for 5 min. The resulting bottom aqueous phase ( ∼ 1.2 ml) was acidified by 25 μl 10 M HCl (to protonate HTPA) and HTPA (and TPA) was extracted (by vortexing) with two 0.9-ml ethyl acetate washes, followed by centrifugation for 5 min at 4,200 g . The combined 1.8 ml ethyl acetate phase was washed with 1.8 ml 0.1 M HCl and evaporated in a rotary vacuum concentrator. The resulting solid precipitate was dissolved in 15 mM KOH (at a minimum volume for example, ∼ 0.1 ml) and adjusted to pH 7 (with 0.2 M KH 2 PO 4 , pH 7) for high-performance liquid chromatography (HPLC) analysis. Samples (10 μl) were injected into an Shimadzu HPLC Prominence UFLC system, consisting of a solvent delivery system (model LC-20AD), a sample manual injector (Rheodyne 7725i), an on-line degasser (DGU-20A5), a reverse-phase C18 column (Waters Nova-Pak C18, 60 Å, 4 μm, 3.9 × 150 mm) and a fluorescent detector (RF-20Axs) set at ex/em 311/425 nm. The mobile phase, consisting of 50 mM KH 2 PO 4 in 30% methanol, pH 3.2 (an alternative mobile phase is 0.2 M KH 2 PO 4 , pH 4.37, containing 2% of KCl [70] ), was passed through the column at a flow rate 0.8 ml min −1 and the sample was eluted for a total of 20 min. HTPA in samples was identified and quantified by HPLC-fluorescence (eluted as a peak at ∼ 14 min) against pure HTPA (article Fig. 1b ), which was synthesized as reported in the Supplementary Methods . HTPA was also identified by mass spectroscopy using an Agilent 1260 Infinity HPLC-MS system equiped with a binary pump, an auto-sampler and a micro-column Zorbax Extend-C18 600Bar 2.1 × 50 mm, 1.8 μM, connected on line with an Agilent 6538 UHD Accurate-Mass Q-TOF LC/MS detector, operated in negative (ESI − ) electrospray ionization mode. Samples (10 μl) were eluted under linear gradient conditions (at a flow rate 0.3 ml min −1 for 10 min) at RT, by an increasing 100% ACN (solvent A) and a decreasing 50 mM KH 2 PO 4 , pH 3.2, 30% MetOH (solvent B) mobile solvent phase. The microcolumn was initially washed with the A and subsequently equilibrated with the solvent B. HTPA (eluted as a peak at ∼ 1.5 min) was identified as giving, for the parent ion, m/z with highest peak at M-1=181.01437 (versus the theoretical 181.01425), and a fragmentation product at M-1=137.02442 (expected from the fragmentation, at CE 20 eV, of one carboxyl group from HTPA). Soil O 2 ·− generation by sunlight and ultraviolet-C Procedure: Soils ( ∼ 1 g), untreated or washed (to remove any soluble inorganics/organics and polar/hydrophobic organics by vortexing (and intermittent centrifugation at 4,200 g for 5 min) with 2 × 10 ml 0.1 M HCl, 1 × 10 ml ddH 2 O, 2 × 10 ml 0.1 M NaOH, 3 × 10 ml ddH 2 O, 2 × 5 ml ddH 2 O plus 5 ml ethyl acetate:ethanol (2:1), 1 × 10 ml 25% ethanol, and finally dried at 150 °C for 1 h) were spread as a thin layer on aluminum foil and exposed to natural sunlight (at 800–1,000 W m −2 , in a July day, from 10:00 to 16:00 hours and at an average 45 °C); unexposed were used as control. The relative humidity at 10:00 hours was ∼ 15% and reached a minimum ∼ 5% during the exposure period. Soils were also exposed to iltraviolet C radiation (using a germicidal lamp with flux density 30 μW cm −2 set at a close distance of 10 cm) at relative humidity 10–25% and at an average 40 °C. After irradiation, soils were extracted for O 2 ·− (as in the Methods section ‘HE-based soil O 2 ·− assay’) and measured by the aforementioned HE-based and SOD-inhibited reduction of cyt. c -based soil O 2 ·− assays. Irradiated soils were also extracted for total superoxides/peroxides and the resulting H 2 O 2 extract was measured as in the Methods section ‘Assay for soil total metal superoxides/peroxides and Fe 3+ ’. Photo-generation of · OH by aqueous desert soils Procedure: Soil samples were extensively washed as in the Methods section ‘Soil O 2 ·− generation by sunlight and ultraviolet C’ to remove any soluble inorganic/organic and polar/hydrophobic organic soil constituents, which may affect the rate of photogeneration of · OH. Washed soil samples (0.2 g) were placed in capped small plastic Petri plates (inner diameter 5 cm), mixed with 10 ml ddH 2 O and spread as an even thin layer on the plate bottom with a small glass rod. Then, 50 μl from the 100 mM TPA stock solution (made in 400 mM NaOH) was added. This resulted in final 0.5 mM TPA and 1 mM NaOH (due to its partial neutralization by the 1 mM carboxyl groups of 0.5 mM TPA), which were set as an optimal for the · OH-TPAassay in a previous study using illuminated TiO 2 films [37] , [38] . Samples were exposed to light irradiation 180 W m −2 (at 400–800 nm, emitted by two halogen lamps, type R7s J118 tube linear 500W/230V ∼ 9000 Lumens per m 2 each, both covered with glass and ultraviolet and infrared cutoff filters and set at 50 cm above the soil plates) or higher (adding more lamps) and for up to 10 h (at RT). The following light-exposed controls were used: (a) soil samples mixed with 10 ml 1 mM NaOH (for soil interference), (b) 10 ml 1 mM NaOH (for aqueous phase treatment interference), (c) 10 ml 0.5 mM TPA and 2 mM NaOH (for TPA interference) ±100 mM DMSO ( · OH scavenger), (d) 10 ml 1 μM H 2 O 2 in 0.5 mM TPA and 2 mM NaOH (to test possible photolysis of H 2 O 2 to · OH; both can be products of, for example, TiO 2 photocatalysis [38] , given that H 2 O 2 can be generated directly or indirectly, for example, via dismutation, from O 2 ·− ) and (e) 10 ml suspension of 1.6 mg TiO 2 (or 20 μM TiO 2 ) in 0.5 mM TPA and 2 mM NaOH (for testing the employed assay to detect · OH photo-generation and by simulating a photocatalysis mechanism with TiO 2 ). The amount of TiO 2 used is equivalent to the average concentration (w%) in the 0.2 g soils from Atacama Yungay and Mojave +CIMA sites ( Table 2 ). Exposure of the soil samples to ultraviolet C irradiation was not used because the control (c) produced · OH, possibly because the ultraviolet C lamp may also emit near the absorbance of water (186 nm) and, thus, photo-dissociate it to · OH. Aqueous samples (1 ml) were drawn from the plates at certain time intervals, centrifuged at 16,000 g for 5 min at RT, acidified with final 0.1 M HCl, extracted × 2 with 1 ml ethyl acetate (by vortexing and subsequent centrifugation at 4,000 g ) and dried by a centrifugal vacuum concentrator at 50 °C. The isolated HTPA solid precipitate in soil and control samples was dissolved in 0.1 ml 20 mM NaOH (its moles are × 2 those of the total carboxy groups of added TPA) and neutralized by 0.2 ml 150 mM K-phosphate buffer, pH 7.4. The solubilized HTPA was quantified by HPLC-fluorescence (as in the Methods section ‘Instability of aqueous desert soil superoxides/peroxides’), and, in routine HTPA quantifications by measuring the fluorescence difference emission spectra (recorded at the excitation wavelength 311 nm) of samples minus those of appropriate controls as follows: Starting with the determination of the emission spectra of controls (a) and (b), they were found identical (indicating that washed soil did not interfere) and lower in FUs than of the control (c) spectrum, which shows that both the controls were part of the control (c). Therefore, the emission spectrum of latter control was subtracted from the soil sample emission spectra taken at different exposure time periods, to estimate the corresponding net emission spectra due to HTPA present in the samples. These HTPA spectra were identified by comparing their shape and peak at 425 nm with the spectra of pure HTPA (synthesized as in the Methods section ‘Instability of aqueous desert soil superoxides/peroxides’), and with the known emission spectra of HTPA, which are stable at a pH range 5.5–9.5 (ref. 70 ). Similarly, the control (c) emission spectrum was subtracted from the emission spectra of controls (d) and (e) to identify the formation of HTPA due to H 2 O 2 and TiO 2 , respectively. The net FU emission peak (at 425 nm with excitation at 311 nm) in the difference spectra was, then, converted to HTPA concentration by a spectrofluorometer (Shimadzu RF-1501) calibrated with 1 μM pure HTPA; it emits ∼ 300 FU at the spectrofluorometer’s low sensitivity setting (or 15,000 FU at the high-sensitivity setting). Additional data analysis is presented in the corresponding section of the Supplementary Methods . Mineralogical and geochemical analysis of soils Procedure: The bulk mineralogy of the samples was determined by X-ray diffraction on the D8 Advance diffractometer (Bruker AXS) equipped with a LynxEye strip silicon detector, using Ni-filtered CuKα radiation, an applied voltage 35 kV and a 35 mA current, and 0.298° divergence and antiscatter slits. The random powder mounts of samples were scanned from 2 to 70° 2 θ with a scanning step of 0.015° 2 θ and with 18.7-s count time per step. Powder diffraction data were collected at RT. Results were confirmed with synchrotron X-ray high-resolution powder diffraction measurements. The samples were loaded into 1.0 mm-diameter glass capillaries. Powder diffraction data (for Atacama Yungay and site 1, and Mojave +CIMA basalt rock samples) were collected at RT (295 K) on the undulator beamline ID31 at the ESRF (European Synchrotron Radiation Facility) in Grenoble, France. The parallel beam geometry instrument is equipped with nine Si(111) analyser crystals and provides data with very high angular resolution, with a minimum instrumental contribution to the full-width half-maximum around 0.003°. High speed spinning of the sample was applied to ensure sufficient powder averaging. The nine detector modules (separated by ∼ 2°) were scanned over a 40° 2 θ range, at a wavelength of 0.400054(15) Å, using an incident beam size of 2.0 mm (2.0 mm (horizontally) × 1.0 mm (vertically)). The clay fraction (<2 μm) was separated by settling and dried on glass slides at RT. Clay minerals were identified from air dried slides and after ethylene glycol solvation at 60 °C overnight to ensure maximum saturation. X-ray diffraction analysis was performed from 2 to 35°2 θ with the Bruker D8 Advance diffractometer, using the same divergence and antiscatter slits, and a step size of 0.019° 2 θ , with 47.7-s count time per step. Chemical composition of minerals was examined with a JEOL 6300 Scanning Electron Microscope equipped with an Oxford Link Energy Dispersive Spectrometer (EDS; Oxford Instruments). Semi-quantitative analyses of minerals were performed on sample powders mounted directly on glass slides and coated with carbon. The chemical composition of the minerals was determined using natural and synthetic standards and 20 kV accelerating voltage with 10 nA beam current. Back-scattered electron images were used to identify any heavy minerals present. The concentrations of major and trace elements in bulk samples (from Atacama sites, Mojave sites and control site) were determined with Energy Dispersive X-ray Florescence Spectroscopy (EDS-XRF, S2 Ranger, Bruker). The samples were fused using a flux:sample powder ratio of 5:1 and were casted in dies forming glass beads. Li-tetraborate was used as flux. Additional data analyses can be found in the corresponding section of the Supplementary Methods . How to cite this article: Georgiou, C. D. et al . Evidence for photochemical production of reactive oxygen species in desert soils. Nat. Commun . 6:7100 doi: 10.1038/ncomms8100 (2015).